Melanoma induction by ultraviolet A but not ultraviolet B radiation requires melanin pigment Malignant melanoma of the skin (CMM) is associated with ultraviolet radiation exposure, but the mechanisms and even the wavelengths responsible are unclear. Here we use a mammalian model to investigate melanoma formed in response to precise spectrally defined ultraviolet wavelengths and biologically relevant doses. We show that melanoma induction by ultraviolet A (320–400 nm) requires the presence of melanin pigment and is associated with oxidative DNA damage within melanocytes. In contrast, ultraviolet B radiation (280–320 nm) initiates melanoma in a pigment-independent manner associated with direct ultraviolet B DNA damage. Thus, we identified two ultraviolet wavelength-dependent pathways for the induction of CMM and describe an unexpected and significant role for melanin within the melanocyte in melanomagenesis. Malignant melanoma of the skin (CMM) is one of the fastest increasing cancers in incidence [1] , [2] . CMM is clearly associated with ultraviolet exposure of genetically susceptible individuals to sunlight or to artificial sources [1] . The epidemiology of melanoma indicates that intermittent, rather than chronic, ultraviolet exposure is a major risk factor for melanoma [3] . Childhood ultraviolet exposure has an important role in melanoma although adult ultraviolet exposure also contributes [4] . Although ultraviolet B is well accepted as a carcinogen for non-melanoma skin cancer, its role in CMM has been controversial [5] and it has been suggested that ultraviolet A, which can initiate different molecular events, may be important [6] , [7] . A role for ultraviolet A in melanoma has, however, also been questioned [8] . The hepatocyte growth factor/scatter factor (HGF) transgenic mouse has provided a model of ultraviolet-induced melanoma [9] , [10] , [11] . The HGF transgenic mouse over-expresses, particularly in melanocytes, the HGF growth factor and HGF signalling pathways are constitutively activated [12] . Notably, the HGF transgenic mouse has ectopic extra-follicular melanocytes in trunk skin at the dermal/epidermal junction and in the epidermis [12] , thus modelling human skin more closely than most animal skin in which melanocytes at these sites are confined to the hair follicle. The HGF transgenic model of ultraviolet melanoma has significant similarities to the pathogenesis of human melanoma and develops, in response to neonatal ultraviolet exposure, melanocytic tumours in stages from early lesions to metastases that are uniquely reminiscent of human cutaneous malignant melanoma [10] , [11] . These include melanomas with pagetoid and junctional histopathology, rare in animal models and not previously found in mouse models. The effectiveness of neonatal ultraviolet irradiation in melanoma development in HGF transgenic mice, confirmed in other mouse models [13] , [14] , is consistent with the critical role for childhood sunlight exposure indicated by epidemiologic studies of human melanoma [4] . The RAS/RAF/MEK/ERK and RAS/PI3K/AKT signalling pathways activated by HGF by its receptor c-MET [15] are highly relevant to melanoma and activating mutations in these pathways, notably in B-RAF or PTEN, occur in a large proportion of human melanomas [16] . MET is an oncogene [17] , [18] , and somatic copy number gains of the C-MET locus are found in almost half of melanomas [19] . Hyperactive c-MET signalling is associated with melanoma progression and metastasis [20] . To unravel the mechanisms by which ultraviolet exposure causes melanoma requires delivery of spectrally defined ultraviolet wavelengths at relevant doses to an appropriate animal model. Here we have used an ultraviolet delivery system designed in our laboratory providing precise control of wavelength and dose delivery [9] together with the HGF transgenic mouse to investigate the roles of ultraviolet B and ultraviolet A in melanoma. We report the existence of two distinct pathways for melanoma: an ultraviolet B initiated, pigment-independent pathway associated with direct ultraviolet B-type DNA damage and an ultraviolet A initiated, pigment-dependent pathway associated with indirect oxidative DNA damage in melanocytes. These studies provide new insights into the mechanistic relationships between cutaneous melanoma and ultraviolet radiation in sunlight and expand the possibilities for development of novel therapeutic approaches. Melanin pigment in melanocytes exacerbates melanoma Three-day-old black or albino HGF littermate pups on a C57BL/6 genetic background (C57BL/6-HGF and C57BL/6-c-HGF respectively) were ultraviolet irradiated as described [9] with a single exposure to 23 standard erythemal doses (SED) or 9.5 kJ m −2 (unweighted) from broadband F40 sunlamps emitting both ultraviolet B and ultraviolet A radiation ( Fig. 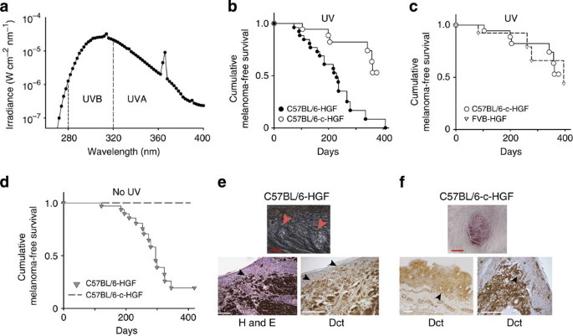Figure 1: Melanoma in ultraviolet-irradiated black and albino HGF transgenic mice. A single melanomagenic dose from F40 sunlamps9,10of 9.5 kJ m−2(23 SED) of ultraviolet radiation containing approximately 65% ultraviolet B and 34% ultraviolet A was delivered to 3-day-old neonatal black C57BL/6-HGF and albino C57BL/6-c-HGF- tyrosinase-mutant pups, which were followed for melanoma development. (a) Ultraviolet (UV) spectral irradiance of F40 sunlamp broadband source. (b) Melanoma in irradiated black C57BL/6-HGF (black circles) and albino C57BL/6-c-HGF (white circles) mice (P<0.001, log-rank test). (c) Melanoma in irradiated albino C57BL/6-c-HGF mice (white circles) compared with previously reported melanoma10in albino FVB-HGF mice irradiated with the same dose of ultraviolet from the same source (white triangles;P=0.9, log-rank test). (d) Melanoma in unirradiated black and albino animals. No spontaneous melanomas occurred in albino C57BL/6-c-HGF mice and spontaneous melanomas arose in black C57BL/6-HGF animals (grey triangles) more slowly than in irradiated mice (P<0.003, log-rank test). (e) Multiple tumours arose in black C57BL/6-HGF mice (red arrows). Pigmented clusters of melanoma cells in the epidermis and at the dermal–epidermal junction (black arrows) were confirmed as melanoma by bleaching and immunohistochemistry for the melanocytic marker Dct. (f) Single tumours that arose in albino C57BL/6-c-HGF mice were invasive into the subcutaneous fat and into the epidermis (black arrows). Red scale bars, 5 mm. White scale bars, 100 μm. 1a , Table 1 ). These ultraviolet doses and wavelengths are highly relevant to human exposure [9] (Methods). We found that the presence of melanin pigment significantly facilitated the development of melanoma. In pigmented animals, melanomas appeared more rapidly than in genetically matched albino animals ( Fig. 1b ), a significantly higher proportion of black than of albino animals produced melanoma and the number of tumours per animal (multiplicity) was increased ( Table 1 ). Comparison of the rates of ultraviolet melanoma formation between the albino C57BL/6-c-HGF strain described here and the genetically distant albino FVB-HGF strain, we previously reported [10] , revealed near identical melanoma response rates, indicating differences in melanoma susceptibility independent of melanin were not a potential confounding effect ( Fig. 1c ). Both albino strains developed melanoma significantly less efficiently in response to F40 irradiation when compared with black C57BL/6-HGF animals. Notably, pigmented C57BL/6-HGF animals also produced spontaneous melanomas (no ultraviolet), which were absent in genetically matched albino C57BL/6-c-HGF transgenic mice ( Fig. 1d ) and were rare in albino FVB-HGF mice [9] . The histology of pigmented and albino melanomas ( Fig. 1e,f ) was comparable to the junctional melanomas, we previously described in neonatally ultraviolet-irradiated albino FVB-HGF mice [10] , [11] . Figure 1: Melanoma in ultraviolet-irradiated black and albino HGF transgenic mice. A single melanomagenic dose from F40 sunlamps [9] , [10] of 9.5 kJ m −2 (23 SED) of ultraviolet radiation containing approximately 65% ultraviolet B and 34% ultraviolet A was delivered to 3-day-old neonatal black C57BL/6-HGF and albino C57BL/6-c-HGF- tyrosinase-mutant pups, which were followed for melanoma development. ( a ) Ultraviolet (UV) spectral irradiance of F40 sunlamp broadband source. ( b ) Melanoma in irradiated black C57BL/6-HGF (black circles) and albino C57BL/6-c-HGF (white circles) mice ( P <0.001, log-rank test). ( c ) Melanoma in irradiated albino C57BL/6-c-HGF mice (white circles) compared with previously reported melanoma [10] in albino FVB-HGF mice irradiated with the same dose of ultraviolet from the same source (white triangles; P =0.9, log-rank test). ( d ) Melanoma in unirradiated black and albino animals. No spontaneous melanomas occurred in albino C57BL/6-c-HGF mice and spontaneous melanomas arose in black C57BL/6-HGF animals (grey triangles) more slowly than in irradiated mice ( P <0.003, log-rank test). ( e ) Multiple tumours arose in black C57BL/6-HGF mice (red arrows). Pigmented clusters of melanoma cells in the epidermis and at the dermal–epidermal junction (black arrows) were confirmed as melanoma by bleaching and immunohistochemistry for the melanocytic marker Dct. ( f ) Single tumours that arose in albino C57BL/6-c-HGF mice were invasive into the subcutaneous fat and into the epidermis (black arrows). Red scale bars, 5 mm. White scale bars, 100 μm. Full size image Table 1 Melanoma in pigmented and albino HGF transgenic mice. Full size table Extra-follicular ectopic melanocytes, absent in wild-type mice but found in HGF transgenic animals ( Fig. 2a ), were present at comparable numbers in albino FVB-HGF and black C57BL/6-HGF transgenic neonatal mouse skin ( Fig. 2b ). Thus, an increase in the number of target melanocytes for potential ultraviolet transformation did not explain the increase in melanoma in pigmented animals. C57BL/6-HGF transgenic neonatal mice could be differentiated from wild-type littermates by a mild hyperpigmentation ( Fig. 2c ). There were only modest increases in skin melanocyte numbers in C57BL/6-HGF neonatal transgenic compared with C57BL/6 wild-type animals (CD45 − c-kit + cells: 2.5% versus 2.0%, respectively, of total skin cells), thus the darker skin in neonatal C57BL/6-HGF transgenics compared with wild-type pups ( Fig. 2c ) appeared to be a result of altered melanocyte distribution, rather than melanocyte number. In contrast to neonates, adult C57BL/6-HGF transgenic animals were grossly hyperpigmented and the skin at all locations appeared black ( Fig. 2c ). In neonatal C57BL/6-HGF transgenic skin, melanin was largely confined to melanocytes where melanosomes were readily distinguishable and there was sparse epidermal pigmentation ( Fig. 2d ). In adult C57BL/6-HGF transgenic skin although epidermal pigment was again sparse, there were clusters of melanocytes, chiefly in the dermis, heavily congested with melanin ( Fig. 2d ). Melanin, determined by electron spin resonance (ESR) in intact skin, consisted of >90% eumelanin and <10% pheomelanin. In both neonatal C57BL/6-HGF transgenic skin and wild-type C57BL/6 skin, constitutive melanin increased by more than twofold from 3 to 5 days of age and levels of melanin were similar between transgenic and wild-type animals ( Fig. 2e ). The density of melanocytes did not increase significantly over this period ( Fig. 2f and ref. 21 ), indicating this increase in melanin in neonatal skin was due to a high activity of pigment synthesis pathways within melanocytes. Adult C57BL/6-HGF transgenic skin had a sixfold higher level of melanin (>90% eumelanin) than adult C57BL/6 wild-type skin ( Fig. 2e ), consistent with the morphological and histological findings and indicating sustained melanin production in adult transgenic but not in wild-type melanocytes. 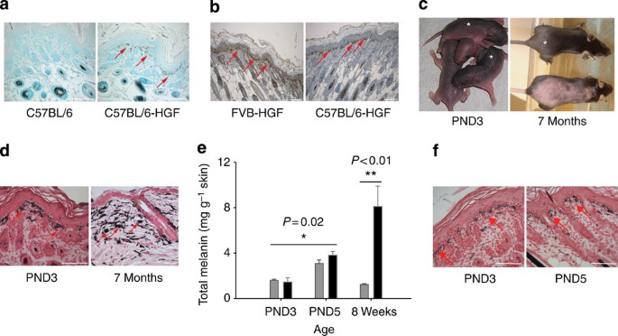Figure 2: Melanocyte and melanin distribution in unirradiated animals. (a) Extra-follicular pigmented cells (arrows) are visible in methyl green-stained skin of 3-day-old C57BL/6-HGF transgenic but not C57BL/6 wild-type mice. (b) Comparable numbers of extra-follicular melanocytes (arrows), visualized by immunohistochemistry for Dct, were observed in skin of 3-day-old albino FVB-HGF and black C57BL/6-HGF mice. Scale bars, 100 μm. (c) Pigmentation of C57BL/6-HGF transgenics (asterisk) and C57BL/6 wild-type littermates (unmarked) at 3 days of age (PND3) and of shaved 7 month old C57BL/6-HGF transgenic mouse (asterisk) compared to shaved wild type animal (unmarked). (d) Melanin (black, Fontana stain) in skin of PND3 and 7-month-old C57BL/6-HGF mice is largely confined to melanocytes and is sparse in the epidermis. Melanosomes were visible in neonatal melanocytes (arrows) but adult (7 months) melanocytes were heavily congested with pigment (arrows). Scale bars, 100 μm. (e) Total melanin in C57BL/6 (grey bars) and C57BL/6-HGF transgenic (black bars) mouse skin determined by ESR was similar between genotypes at each neonatal time point (P>0.1,t-test) but increased significantly in both genotypes between PND3 and PND5 (*t-test). Adult HGF transgenic skin (8 weeks) had more than sixfold the melanin of adult wild-type skin (**t-test). Bars represent mean±s.e.m. of 3–5 biological replicates. No melanin was detectable in albino skin. (f) Frequencies of extra-follicular melanocytes (arrows) are similar in 3- and 5-day-old (PND5) neonatal C57BL/6-HGF skin. Fontana stain. Scale bars, 100 μm. Figure 2: Melanocyte and melanin distribution in unirradiated animals. ( a ) Extra-follicular pigmented cells (arrows) are visible in methyl green-stained skin of 3-day-old C57BL/6-HGF transgenic but not C57BL/6 wild-type mice. ( b ) Comparable numbers of extra-follicular melanocytes (arrows), visualized by immunohistochemistry for Dct, were observed in skin of 3-day-old albino FVB-HGF and black C57BL/6-HGF mice. Scale bars, 100 μm. ( c ) Pigmentation of C57BL/6-HGF transgenics (asterisk) and C57BL/6 wild-type littermates (unmarked) at 3 days of age (PND3) and of shaved 7 month old C57BL/6-HGF transgenic mouse (asterisk) compared to shaved wild type animal (unmarked). ( d ) Melanin (black, Fontana stain) in skin of PND3 and 7-month-old C57BL/6-HGF mice is largely confined to melanocytes and is sparse in the epidermis. Melanosomes were visible in neonatal melanocytes (arrows) but adult (7 months) melanocytes were heavily congested with pigment (arrows). Scale bars, 100 μm. ( e ) Total melanin in C57BL/6 (grey bars) and C57BL/6-HGF transgenic (black bars) mouse skin determined by ESR was similar between genotypes at each neonatal time point ( P >0.1, t -test) but increased significantly in both genotypes between PND3 and PND5 (* t -test). Adult HGF transgenic skin (8 weeks) had more than sixfold the melanin of adult wild-type skin (** t -test). Bars represent mean±s.e.m. of 3–5 biological replicates. No melanin was detectable in albino skin. ( f ) Frequencies of extra-follicular melanocytes (arrows) are similar in 3- and 5-day-old (PND5) neonatal C57BL/6-HGF skin. Fontana stain. Scale bars, 100 μm. Full size image Ultraviolet B and Ultraviolet A dependence of melanoma As we had identified a major effect of melanin on melanoma using a broadband ultraviolet source, which emitted both ultraviolet B and ultraviolet A, we next sought to establish which of these spectral regions was responsible for the effect. We previously found in albino FVB-HGF mice that ultraviolet B but not ultraviolet A initiated melanoma [9] . Using the same specialized ultraviolet sources and doses [9] , black C57BL/6-HGF neonates were irradiated with a single exposure to either spectrally defined ultraviolet B (>98% 280–320 nm) or spectrally defined ultraviolet A (>99% 320–400 nm) radiation ( Fig. 3a ) and melanoma formation was assessed ( Fig. 3b ). As previously described [9] , [21] , the doses of ultraviolet B and ultraviolet A were biologically relevant (Methods) and could have been readily received in summer sunlight [22] . The absolute ultraviolet B dose delivered was more than tenfold less than the ultraviolet A dose ( Table 1 ) and approximated the ultraviolet B/A ratios in sunlight where ultraviolet A is more abundant [9] . As expected, ultraviolet B was highly melanomagenic but, in contrast to the previous data for albino mice, ultraviolet A treatment of pigmented animals also initiated melanoma ( Fig. 3b ). Ultraviolet B was significantly more effective at melanomagenesis than ultraviolet A and melanomas arose significantly faster in both ultraviolet-irradiated groups than in unirradiated animals ( Fig. 3b , Table 1 ). 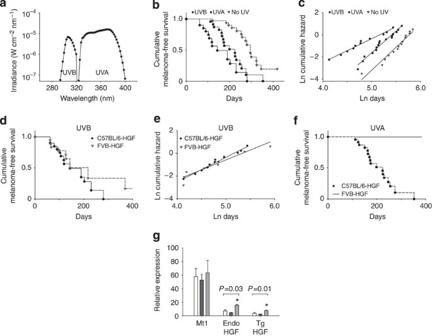Figure 3: Melanoma initiated by spectrally isolated ultraviolet B and ultraviolet A (UVB and UVA). (a) Spectral irradiance of ultraviolet sources. Ultraviolet delivered as a single dose to neonatal mice was 14 kJ m−2of ultraviolet B (>98%, 280–320 nm) or 150 kJ m−2of ultraviolet A radiation (>99%, 320–400 nm). (b) Melanomas initiated by ultraviolet B, ultraviolet A and spontaneous melanomas (no ultraviolet) in C57BL/6-HGF mice were significantly different by log-rank test (P<0.001). Pairwise comparisons: ultraviolet B versus no ultraviolet,P<0.001, ultraviolet A versus no ultraviolet,P=0.001, log-rank test; ultraviolet A versus B,P=0.02, Gehan–Wilcoxon test. (c) Log transform of data in panelb. The slope of the line for ln cumulative hazard as a function of ln days for ultraviolet B was significantly different from the slopes for ultraviolet A or for no ultraviolet,P<2×10−5. Slopes for ultraviolet A and no ultraviolet were similar (P=0.5), but intercepts were significantly different (P=4×10−12). Analysis by ANOVA with Tukeypost-hoctest for multiple comparisons. (d) Melanoma in ultraviolet B irradiated black C57BL/6-HGF and albino FVB-HGF transgenic mice was similar (P=0.3, log-rank test). (e) Log transform of data in paneld. There was no significant difference between the slopes (P=0.4) or the intercepts (P>0.08) for the two strains. Statistical analysis as for panelc. (f) Ultraviolet A irradiation resulted in melanomas in black C57BL/6-HGF but not in albino FVB-HGF transgenics. Data in panelbfor unirradiated animals is fromFig. 1b. Data in paneldand panelffor FVB-HGF animals were previously published9. (g) Real-time quantitative PCR was performed on back skin samples of untreated (no ultraviolet, white bars), ultraviolet A (black bars) and ultraviolet B (grey bars)-treated C57BL/6-HGF neonates, 24 h after irradiation with doses of 14 kJ m−2of ultraviolet B or 150 kJ m−2of ultraviolet A. Data are mean±s.e.m. from four (no ultraviolet, ultraviolet A) or three (ultraviolet B) biological replicates. Neither ultraviolet B nor ultraviolet A significantly affected expression of endogenous Mt1 (P=0.7). Ultraviolet A did not affect expression of either transgenic (P=0.2) or endogenous (P=0.19) HGF. Ultraviolet B significantly increased expression of both transgenic and endogenous HGF compared with corresponding no ultraviolet samples, indicating an Mt1-independent mechanism. Statistical analyses performed by two-way ANOVA test. Figure 3: Melanoma initiated by spectrally isolated ultraviolet B and ultraviolet A (UVB and UVA). ( a ) Spectral irradiance of ultraviolet sources. Ultraviolet delivered as a single dose to neonatal mice was 14 kJ m −2 of ultraviolet B (>98%, 280–320 nm) or 150 kJ m −2 of ultraviolet A radiation (>99%, 320–400 nm). ( b ) Melanomas initiated by ultraviolet B, ultraviolet A and spontaneous melanomas (no ultraviolet) in C57BL/6-HGF mice were significantly different by log-rank test ( P <0.001). Pairwise comparisons: ultraviolet B versus no ultraviolet, P <0.001, ultraviolet A versus no ultraviolet, P =0.001, log-rank test; ultraviolet A versus B, P =0.02, Gehan–Wilcoxon test. ( c ) Log transform of data in panel b . The slope of the line for ln cumulative hazard as a function of ln days for ultraviolet B was significantly different from the slopes for ultraviolet A or for no ultraviolet, P <2×10 −5 . Slopes for ultraviolet A and no ultraviolet were similar ( P =0.5), but intercepts were significantly different ( P =4×10 −12 ). Analysis by ANOVA with Tukey post-hoc test for multiple comparisons. ( d ) Melanoma in ultraviolet B irradiated black C57BL/6-HGF and albino FVB-HGF transgenic mice was similar ( P =0.3, log-rank test). ( e ) Log transform of data in panel d . There was no significant difference between the slopes ( P =0.4) or the intercepts ( P >0.08) for the two strains. Statistical analysis as for panel c . ( f ) Ultraviolet A irradiation resulted in melanomas in black C57BL/6-HGF but not in albino FVB-HGF transgenics. Data in panel b for unirradiated animals is from Fig. 1b . Data in panel d and panel f for FVB-HGF animals were previously published [9] . ( g ) Real-time quantitative PCR was performed on back skin samples of untreated (no ultraviolet, white bars), ultraviolet A (black bars) and ultraviolet B (grey bars)-treated C57BL/6-HGF neonates, 24 h after irradiation with doses of 14 kJ m −2 of ultraviolet B or 150 kJ m −2 of ultraviolet A. Data are mean±s.e.m. from four (no ultraviolet, ultraviolet A) or three (ultraviolet B) biological replicates. Neither ultraviolet B nor ultraviolet A significantly affected expression of endogenous Mt1 ( P =0.7). Ultraviolet A did not affect expression of either transgenic ( P =0.2) or endogenous ( P =0.19) HGF. Ultraviolet B significantly increased expression of both transgenic and endogenous HGF compared with corresponding no ultraviolet samples, indicating an Mt1-independent mechanism. Statistical analyses performed by two-way ANOVA test. Full size image The Kaplan–Meier survival data from Fig. 3b were log–log transformed to obtain linear plots ( Fig. 3c ). The slope of the log–log transformed plot for melanoma initiated by ultraviolet B was significantly different from that for melanoma initiated by ultraviolet A (ultraviolet B: 2.2±0.08; ultraviolet A: 3.9±0.2, P <2×10 −5 ; analysis of variance (ANOVA) with Tukey post-hoc test for multiple comparisons) prompting us to hypothesize that different mechanisms could be responsible for initiation of melanoma by ultraviolet B and ultraviolet A. A difference in mechanism was supported when the effectiveness of initiating melanoma by ultraviolet B or ultraviolet A was compared between the black C57BL/6-HGF strain reported here and the previously published data for the albino FVB-HGF strain [9] ( Fig. 3d–f ). For ultraviolet B, the rate of melanoma appearance was not significantly different between black C57BL/6-HGF and albino FVB-HGF mice ( Fig. 3d ) and the slopes and intercepts of the log–log transformed plots were also similar ( Fig. 3e ). Thus, the initiation of melanoma by ultraviolet B was pigment independent. In contrast, melanoma induction by ultraviolet A was completely pigment dependent. Melanomas were initiated by ultraviolet A in black C57BL/6-HGF transgenics but no melanomas were seen in ultraviolet A-irradiated albino FVB-HGF mice ( Fig. 3f ). Ultraviolet A-induced melanoma was not a result of increased transgene HGF expression driven by oxidative effects on the metallothionein transgene promoter, as metallothionein (Mt1), transgenic HGF and endogenous HGF expression were not altered in neonatal skin by ultraviolet A irradiation ( Fig. 3g ). DNA damage in response to ultraviolet B and ultraviolet A The existence of two wavelength-dependent mechanisms for ultraviolet-induced melanoma was further supported by examination of DNA damage in skin from ultraviolet-irradiated neonatal mice. Cyclobutane pyrimidine dimers (CPDs) were readily detectable by immunohistochemistry in albino FVB-HGF and black C57BL/6-HGF skins irradiated with ultraviolet B but not in skin irradiated with ultraviolet A ( Fig. 4a ). CPDs and 6-4 photoproducts (6-4PPs) quantified by high-performance liquid chromatography-tandem mass spectroscopy (HPLC-MS/MS) were comparable in albino FVB-HGF and black C57BL/6-HGF animals after ultraviolet B irradiation ( Fig. 4b ). In contrast, after ultraviolet A irradiation, in both strains, only TT-CPD lesions were detected but at greatly reduced levels compared with ultraviolet B-irradiated animals and no 6-4PPs were found ( Fig. 4b ), in accordance with previous studies [23] . Ultraviolet A-induced levels of TT-CPDs in C57BL/6-HGF skin were similar to those in FVB-HGF skin ( Fig. 4b ), indicating that ultraviolet A-induced CPD formation could not explain the difference in melanoma induction between pigmented and albino animals. 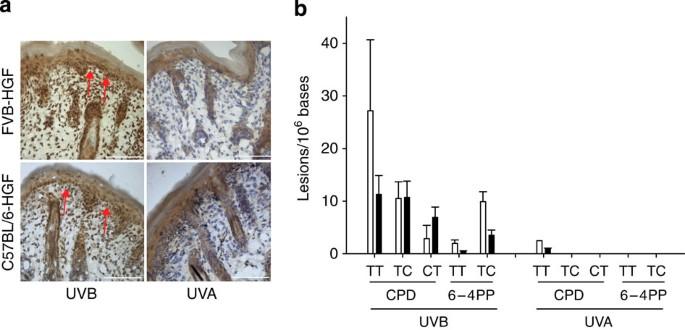Figure 4: Ultraviolet B induced DNA damage in neonatal skin. (a) Immunohistochemistry for CPD DNA damage (brown nuclei) in skin from neonatal FVB-HGF and C57BL/6-HGF transgenic mice irradiated with ultraviolet B (14 kJ m−2) or ultraviolet A (150 kJ m−2). Arrows indicate nuclear CPDs at the dermal/epidermal junction. No CPDs were detected in ultraviolet A irradiated skin (blue nuclei). Scale bar, 100 μm. (b) CPD and 6-4PP lesions quantified in skin extracts by HPLC-MS/MS from FVB-HGF (white bars) and C57BL/6-HGF (black bars) transgenic mice ultraviolet irradiated as in panela. Values are mean±s.e.m. of triplicate biological replicates. No CPD or 6-4PP lesions were detected in unirradiated skin of either strain. Figure 4: Ultraviolet B induced DNA damage in neonatal skin. ( a ) Immunohistochemistry for CPD DNA damage (brown nuclei) in skin from neonatal FVB-HGF and C57BL/6-HGF transgenic mice irradiated with ultraviolet B (14 kJ m −2 ) or ultraviolet A (150 kJ m −2 ). Arrows indicate nuclear CPDs at the dermal/epidermal junction. No CPDs were detected in ultraviolet A irradiated skin (blue nuclei). Scale bar, 100 μm. ( b ) CPD and 6-4PP lesions quantified in skin extracts by HPLC-MS/MS from FVB-HGF (white bars) and C57BL/6-HGF (black bars) transgenic mice ultraviolet irradiated as in panel a . Values are mean±s.e.m. of triplicate biological replicates. No CPD or 6-4PP lesions were detected in unirradiated skin of either strain. Full size image As ultraviolet A is known to induce DNA damage indirectly through photooxidative mechanisms, we investigated oxidative DNA damage in neonatal skin and in cultured melanocytes. 8-Oxo-7,8-dihydro-2′-deoxyguanosine (8-oxodGuo) was detected in the nuclei of extra-follicular melanocytes at the dermal/epidermal junction in neonatal skin after ultraviolet A irradiation of pigmented C57BL/6-HGF mice but not of albino FVB-HGF mice ( Fig. 5a,b ). Quantification of staining intensity identified a major population of cells with significantly increased intensity of nuclear 8-oxodGuo staining (>20 units of pixel intensity Fig. 5c ). These were found only in skin from ultraviolet A-irradiated pigmented C57BL/6-HGF neonates after ultraviolet A irradiation and not in skin from unirradiated black animals or in skin from albino animals with or without ultraviolet A irradiation. Ultraviolet B, in contrast, was very poorly effective at initiating nuclear 8-oxodGuo in pigmented C57BL/6-HGF melanocytes in neonatal skin ( Fig. 5d,e ). The increased 8-oxodGuo in response to ultraviolet A was due to the presence of melanin and not to genetic differences between mouse strains as ultraviolet A-irradiated albino C57BL/6-c animals had very low levels of nuclear 8-oxodGuo ( Fig. 5f,g ). Scoring for nuclear 8-oxodGuo staining in melanocytes, which were identified by the presence of cytoplasmic melanin, found that >95% of melanocyte nuclei in ultraviolet A-irradiated black C57BL/6-HGF skin exhibited >20 units of pixel intensity, indicating prominent DNA photoxidation in pigmented melanocytes ( Fig. 5h ). Nuclear 8-oxodGuo was also significantly increased in cultured black pigmented melanocytes (Melan-a) but not in albino melanocytes (Melan-c) after irradiation with ultraviolet A ( Fig. 5i ), further confirming a photooxidative interaction between ultraviolet A and melanin in melanocytes. 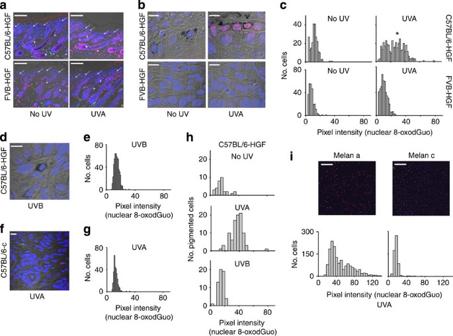Figure 5: Ultraviolet A induced oxidative DNA damage in neonatal skin and cultured melanocytes. (a) Extra-follicular melanocytes (arrows) show increased nuclear 8-oxodGuo (pink) after 150 kJ m−2of ultraviolet A in C57BL/6-HGF but not in FVB-HGF skin. Nuclear 8-oxodGuo is visible in all panels in the hair follicle outer root sheath (white arrowheads) and in the hair bulb of C57BL/6-HGF-pigmented skin where it is increased by ultraviolet A (asterisks) but is sparse in the hair bulb of albino FVB-HGF skin. Green arrowheads, autofluorescence. Scale bars, 150 μm. (b) Oxidative DNA damage in cell nuclei at the dermal–epidermal junction is present in pigmented C57BL/6-HGF but not in albino FVB-HGF skin after ultraviolet A (150 kJ m−2). Scale bars, 10 μm. (c) Histogram of nuclear 8-oxodGuo (Volocity software analysis) of high-power confocal images of epidermal–dermal junctional skin. Nuclei counted (n) in C57BL/6-HGF: no ultraviolet 236, ultraviolet A 397; FVB-HGF: no ultraviolet 253, ultraviolet A 476. Comparison between four groups,P<0.001 (Kruskal–Wallis); all pairwise comparisonsP<0.05 (Dunn's method). Significant nuclear 8-oxodGuo pixel intensity >20 arbitrary units (asterisk) is apparent only in ultraviolet A-irradiated C57BL/6-HGF skin. (d,e) Ultraviolet B (14 kJ m−2) was ineffective compared with ultraviolet A, at producing nuclear 8-oxodGuo in C57BL/6-HGF skinP<0.001 , Mann-Whitney. (Histogram,n=550). Scale bar, 10 μm. (f,g) Albino C57BL/6-c mice are not susceptible to nuclear 8-oxodGuo induction by ultraviolet A (150 kJ m−2), significantly different from nuclear 8-oxodGuo in ultraviolet A-irradiated C57BL/6-HGF skin,P<0.001, Mann–Whitney. (Histogram,n=300). Scale bar, 10 μm. Green is autofluorescence. (h) Neonatal pigmented melanocytes produce 8-oxodGuo in response to ultraviolet A (150 kJ m−2) but not to ultraviolet B (14 kJ m−2). Nuclear 8-oxodGuo was quantified as in panelc, but only in pigmented extra-follicular melanocytes, identified by the presence of black cytoplasmic melanin. 8-OxodGuo was significantly increased in C57BL/6-HGF melanocytes (n=92) after ultraviolet A, compared with no ultraviolet (n=32) or to ultraviolet B (n=57),P<0.001, Kruskal–Wallis. (i) Ultraviolet A irradiated (1.35 kJ m−2) cultured pigmented Melan-a melanocytes produce more 8-oxodGuo than albino Melan-c melanocytes. Scale bar, 250 μm. Histograms: 8-oxodGuo in Melan-a (n=524) compared with Melan-c (n=576),P<0.001, Mann–Whitney. 8-OxodGuo in unirradiated Melan-c or Melan-a cells (n>350 per cell line) was <6 units. Ultraviolet A dose was not phototoxic. Figure 5: Ultraviolet A induced oxidative DNA damage in neonatal skin and cultured melanocytes. ( a ) Extra-follicular melanocytes (arrows) show increased nuclear 8-oxodGuo (pink) after 150 kJ m −2 of ultraviolet A in C57BL/6-HGF but not in FVB-HGF skin. Nuclear 8-oxodGuo is visible in all panels in the hair follicle outer root sheath (white arrowheads) and in the hair bulb of C57BL/6-HGF-pigmented skin where it is increased by ultraviolet A (asterisks) but is sparse in the hair bulb of albino FVB-HGF skin. Green arrowheads, autofluorescence. Scale bars, 150 μm. ( b ) Oxidative DNA damage in cell nuclei at the dermal–epidermal junction is present in pigmented C57BL/6-HGF but not in albino FVB-HGF skin after ultraviolet A (150 kJ m −2 ). Scale bars, 10 μm. ( c ) Histogram of nuclear 8-oxodGuo (Volocity software analysis) of high-power confocal images of epidermal–dermal junctional skin. Nuclei counted ( n ) in C57BL/6-HGF: no ultraviolet 236, ultraviolet A 397; FVB-HGF: no ultraviolet 253, ultraviolet A 476. Comparison between four groups, P <0.001 (Kruskal–Wallis); all pairwise comparisons P <0.05 (Dunn's method). Significant nuclear 8-oxodGuo pixel intensity >20 arbitrary units (asterisk) is apparent only in ultraviolet A-irradiated C57BL/6-HGF skin. ( d , e ) Ultraviolet B (14 kJ m −2 ) was ineffective compared with ultraviolet A, at producing nuclear 8-oxodGuo in C57BL/6-HGF skin P <0.001 , Mann-Whitney. (Histogram, n =550). Scale bar, 10 μm. ( f , g ) Albino C57BL/6-c mice are not susceptible to nuclear 8-oxodGuo induction by ultraviolet A (150 kJ m −2 ), significantly different from nuclear 8-oxodGuo in ultraviolet A-irradiated C57BL/6-HGF skin, P <0.001, Mann–Whitney. (Histogram, n =300). Scale bar, 10 μm. Green is autofluorescence. ( h ) Neonatal pigmented melanocytes produce 8-oxodGuo in response to ultraviolet A (150 kJ m −2 ) but not to ultraviolet B (14 kJ m −2 ). Nuclear 8-oxodGuo was quantified as in panel c , but only in pigmented extra-follicular melanocytes, identified by the presence of black cytoplasmic melanin. 8-OxodGuo was significantly increased in C57BL/6-HGF melanocytes ( n =92) after ultraviolet A, compared with no ultraviolet ( n =32) or to ultraviolet B ( n =57), P <0.001, Kruskal–Wallis. ( i ) Ultraviolet A irradiated (1.35 kJ m −2 ) cultured pigmented Melan-a melanocytes produce more 8-oxodGuo than albino Melan-c melanocytes. Scale bar, 250 μm. Histograms: 8-oxodGuo in Melan-a ( n =524) compared with Melan-c ( n =576), P <0.001, Mann–Whitney. 8-OxodGuo in unirradiated Melan-c or Melan-a cells ( n >350 per cell line) was <6 units. Ultraviolet A dose was not phototoxic. Full size image We report here the identification of two ultraviolet wavelength-dependent pathways associated with the induction of CMM. Ultraviolet B was more effective than ultraviolet A at initiating melanoma, reinforcing the view that ultraviolet B is a major factor in melanoma initiation [9] and reviewed in ref. 5 . CPDs are the predominant ultraviolet B lesion in DNA as confirmed here and can result, if unrepaired, in C to T and CC to TT transition ultraviolet B-type mutations [24] , which have been closely associated with non-melanoma skin cancer, but have been elusive in melanoma [5] although ultraviolet B mutations have been reported in melanomas from human subjects with the DNA repair deficiency xeroderma pigmentosum [25] . Two recent studies in which the genomes of human melanomas were sequenced found a majority of the mutations to have ultraviolet B signatures, further supporting the relevance of our observations to human melanoma [26] , [27] . In contrast to ultraviolet B, we found that CPD formation could not explain ultraviolet A-induced melanoma. TT-CPDs occurred with very low frequency after ultraviolet A irradiation of neonatal skin and the presence of melanin did not enhance their formation. Ultraviolet A melanoma was instead associated with oxidative DNA damage. We detected what is considered the most abundant oxidative product in ultraviolet A-induced DNA damage, 8-oxodGuo [24] , in the nuclei of pigmented melanocytes in ultraviolet A irradiated neonatal skin. This production of 8-oxodGuo oxidative DNA damage required both ultraviolet A radiation and the presence of melanin. 8-OxodGuo is highly mutagenic and can result in G-C to T-A transversion mutations, which are considered signature lesions for reactive oxygen species (ROS)-type DNA damage [24] . The concept that ultraviolet A initiates melanoma in the HGF mouse model through an oxidative process is consistent with the reported effectiveness of the anti-oxidant N -acetyl cysteine in decreasing melanoma in HGF transgenic mice irradiated with a broadband ultraviolet sunlamp with an emission spectrum similar to that in Fig. 1a [28] . ROS-type mutations, originating predominantly from oxidized guanine, were the second most common mutations sequenced in a human melanoma, further supporting a role for oxidative processes in the pathogenesis of this human disease [27] . Melanin in the C57BL/6-HGF mouse consists of >90% eumelanin. Black eumelanin is a complex heterogeneous polymer of 5,6-dihydroxyindole and 5,6-dihydroxyindole-2-carboxylic acid and their derivatives [29] and has opposing properties. It can be an excellent optical absorber, anti-oxidant and free-radical scavenger, but, on absorption of radiation can form melanin radicals which, particularly in the presence of redox-active metal ions, are strong oxidants [29] , [30] , [31] . Partially polymerized melanin is more effective in photooxidation than is fully aggregated melanin [32] and melanin synthesis, which we have shown to be very active in our melanoma mouse model, proceeds through a series of highly reactive quinone intermediates that promote the production of ROS and oxidative DNA damage [33] , [34] . Ultraviolet A can interact oxidatively with these melanin precursors to produce polymerized melanin [35] , [36] . Ultraviolet A irradiation of melanin-containing human melanocytes was reported to promote oxidative DNA damage, which was exacerbated by stimulation of pigment synthesis before irradiation [37] . It has recently been reported that human melanocytes have deficient repair of oxidative DNA damage, proposed to result from melanin interference with DNA repair processes [38] , further emphasizing the vulnerability of pigmented melanocytes to ultraviolet A photooxidation. Additional mechanistic studies are required to establish that oxidation products in melanocytes are the critical ultraviolet A lesions for melanoma development and to understand the relative roles of oxidative DNA damage and of processes resulting from cellular oxidative stress including epigenetic alterations (reviewed in ref. 39 ). As ultraviolet A activates multiple cellular signalling pathways [40] , it may also have a tumour promotional role in pigment-dependent melanomagenesis. An unanticipated observation was that black C57BL/6-HGF mice produced spontaneous melanomas without ultraviolet exposure, although spontaneous melanomas were not found in albino C57BL/6-c-HGF transgenic mice and were rare in albino FVB-HGF mice [9] . A potential confounding melanomagenic effect from ambient lighting was eliminated when the experiment was repeated in a light environment devoid of any ultraviolet radiation. Under these conditions, both ultraviolet B- and ultraviolet A-induced and spontaneous tumours arose at similar rates to those originally observed, eliminating this possibility. Although ultraviolet A tumours arose more rapidly than spontaneous tumours in black C57BL/6-HGF mice, the slopes of the log–log transformed plots for ultraviolet A and for spontaneous tumours were similar ( Fig. 3c ), consistent with the fact that both were dependent on the presence of melanin, suggesting similar mechanisms. We observed that C57BL/6-HGF melanocytes became progressively hyperpigmented and congested with melanin with age. Disturbed melanin synthesis in dysplastic nevi has been associated with enhanced oxidative stress [30] , [34] . Taking these observations together, we hypothesize that endogenous oxidation by dysregulated melanin biosynthesis is responsible for the melanomas in unirradiated animals and contributes to the increased melanoma multiplicity in all pigmented groups. These findings suggest an ultraviolet-independent role for dysregulated melanogenesis in human melanoma and raise the question of whether endogenous oxidation by dysregulated melanogenesis may be a contributor to the development of rare human melanomas in non-sun-exposed sites such as the mucosal melanomas found in ano-rectal or oesophageal melanoma [41] . Disorganization of melanin synthesis is frequently observed in melanoma [42] . Notably, high levels of melanin pigment have been proposed as one of the diagnostic criteria specifically for human B-RAF mutant melanoma [43] . Activation of β-catenin in a genetically engineered melanoma-susceptible mouse model expressing the B-RAFV600E human mutation together with melanocyte-specific Pten loss resulted in uniform melanoma hyperpigmentation and a more aggressive phenotype [44] . We would note that use of unregulated superpotent peptide tanning agents that hyperstimulate pigment synthesis have been reported to result in atypical nevi [45] and melanoma [46] , further supporting the potential adverse effects of hyperpigmentation. Further investigations are required to firmly establish which mechanisms are responsible. An adverse role for melanin in melanoma may appear to run counter to the concept that melanin is protective [2] , [47] . Constitutive skin colour is, however, attained in a series of well regulated, ultraviolet-independent processes, which include melanin synthesis and result in arrangement of melanosomes in an ultraviolet-protective configuration within epidermal cells [48] . These processes are highly effective in darker skin where the constitutive epidermal melanin has been shown not only to confer the dark skin colour but also to screen successfully the underlying melanocytes from ultraviolet damage [47] . In constitutively fair skin, these processes are much less effective, and the resulting epidermal pigmentation is much less protective [47] , leaving the melanocytes vulnerable to direct absorption of ultraviolet radiation—as happens in the C57BL/6-HGF mouse model. Skin responds to ultraviolet exposure with protective responses, which include facultative pigmentation (or tanning). In contrast to constitutive pigmentation, however, a tan is a relatively poor protector against subsequent ultraviolet damage and tanning in response to ultraviolet A conferred no protection [36] . Our studies suggest, therefore, that minimally protected melanocytes in fair skin are vulnerable not only to ultraviolet B but, if stimulated to carry out melanin synthesis, are also vulnerable to ultraviolet A-induced melanoma. Consistent with this, nevi at exposed sites progressed to severe dysplasia and to melanoma following a series of sunbed exposures that induced tanning (Tucker M., unpublished data and ref. 49 ), arguing against the idea that sunbed-induced tanning offers protection against skin cancer. The model we have derived for melanoma, using precisely defined ultraviolet sources and a relevant genetically engineered mouse, has provided several novel and compelling insights potentially applicable to human melanoma. Here we confirm the importance of ultraviolet B in melanoma, particularly significant in view of the increasing melanoma incidence rates and the potential health effects [50] of global increases in ultraviolet B directly associated with stratospheric ozone depletion over highly populated latitudes [51] . We further provide evidence for a novel and important role of ultraviolet A in concert with melanin in melanoma and thus provide an experimental explanation for the observations that artificial ultraviolet A tanning is a significant melanoma risk [52] particularly in young women [53] . Notably, the ultraviolet A doses used in this study could be received from an average tanning bed in 6–12 min (ref. 54 ). Our experimental findings of an important role for dysregulated melanin in melanoma is provocative given that the presence of pigmented nevi is the strongest genetic risk factor for melanoma [1] . Finally, these observations provide at least a partial explanation for the well-described conundrum that African albinos, who have melanocytes but lack melanin, are highly susceptible to non-melanoma skin cancer but are relatively resistant to cutaneous malignant melanoma [55] , [56] . In summary, the demonstration of pigment-independent ultraviolet B and pigment-dependent ultraviolet A pathways in mammalian melanoma is novel and is expected to lead to deeper insights into the mechanisms of melanoma formation by solar ultraviolet radiation. Ultraviolet irradiation Neonatal pups were ultraviolet irradiated with a single dose of ultraviolet at 3 days of age. The ultraviolet doses used caused occasional mild desquamation and no inflammatory neutrophil infiltrate [9] , [10] , [11] , [21] , [57] . Initially, a dose of ultraviolet radiation of 9.5 kJ m −2 from a bank of six F40 sunlamps, corresponding to 23 SED [9] , [10] , [21] was used. Subsequently, a customized optical source was used that coupled ultraviolet interference or cutoff filters to a 2.5-kW xenon arc light system to produce isolated ultraviolet B or isolated ultraviolet A [9] . The spectrally defined ultraviolet B source coupled a ultraviolet B bandpass interference filter (HBW ±5 nm; size: 5.08×5.08 cm 2 ; blocked 10 −3 to 10 −4 outside the main bandpass (280–320 nm)) from X-ray to the far infrared and the spectrally defined ultraviolet A source coupled a ultraviolet A bandpass interference filter (HBW ±40 nm; size: 5.08×5.08 cm 2 ; blocked 10 −3 to 10 −4 from X-ray to the far infrared outside the main bandpass (320–400 nm)) to the xenon arc light system. Average beam irradiance was measured with an Optronics 742 spectroradiometer (Optronics, Orlando, FL). Five different spectroradiometer positions were used within the beam field, before and/or after each experiment. Both an absolute irradiance and an erythemally effective irradiance were determined [9] , [21] . An 0.30–0.32 CIE-erythemally effective W m −2 irradiance was produced for ultraviolet B exposure. The ultraviolet B exposure time was adjusted to produce a CIE-effective dose of 23 SED. The absolute ultraviolet B dose delivered was 14 kJ m −2 (unweighted). Direct measurements on human subjects indicate that under summer sunlight in the mid-latitudes of the Northern Hemisphere, SEDs in the range of 10 to 20 depending on exposure conditions [22] can be readily received. For ultraviolet A exposure, it was necessary to use an unweighted rather than a biologically effective dose [9] because ultraviolet A is much less effective than ultraviolet B in producing erythema. Exposure from the spectrally defined ultraviolet A waveband (>99.9%, 320–400 nm) was 150 kJ m −2 . This dose of ultraviolet A could be received in mid-summer at Northern mid-latitudes, clear sky in approximately 50 min between 1100 and 1500 hours (ref. 9 ). Mice C57BL/6NCr, FVB/N and C57BL/6-cBrd/cBrd/Cr breeding animals were supplied by the National Cancer Institute, Frederick, MD. C57BL/6NCr-HGF/SF (designated C57BL/6-HGF), C57BL/6-cBrd/cBrd/Cr-HGF/SF (designated C57BL/6-c-HGF) and FVB/N-HGF/SF (designated FVB-HGF) transgenic animals were bred at the George Washington University. For the first series of studies, C57BL/6-HGF males and C57BL/6-c females were bred and the resulting F1 HGF transgenic males backcrossed with C57BL/6-c females. Black and albino wild-type and HGF transgenic littermates from this backcross were irradiated with F40 sunlamps and followed for melanoma formation. In other experiments, C57BL/6-HGF animals were irradiated with specialized sources of ultraviolet B and A described above. All experiments were carried out with Institutional Animal Care and Use Committee approval and according to the National Institutes of Health guidelines for animal care and use. Melanoma observations Animals were shaved at 2 months of age and monitored every 2 weeks for skin lesion development [9] , [10] . For survival analysis, time to first lesion subsequently confirmed as a melanoma was used. All melanomas were histologically confirmed [9] , [10] . Non-melanoma skin cancers were not observed. A minority of animals developed hepatocellular adenomas or occasionally spontaneous lung alveolar carcinomas. Histology and immunohistochemistry Skin sections: pigment was visualized in skin sections using methyl green or Fontana stain. Melanocytes were visualized using a primary antibody to Dct and peroxidase-labelled secondary antibody with diaminobenzidine (DAB) [11] . CPDs were detected by immunohistochemistry [57] . For detection of oxidative DNA damage, skin samples harvested at 10 min post ultraviolet irradiation were fixed in 4% phosphate-buffered paraformaldehyde. Sections were treated with DNase-free RNase A (5 mg ml −1 in tris-buffered saline (TBS)), antigen retrieval performed in citrate buffer (pH 6). Sections were blocked with Mouse-on-Mouse (M.O.M.) blocking reagent (Vector Laboratories) and were stained with Clone N45.1 antibody 5 mg/ml in M.O.M. diluent (Japan Institute for the Control of Aging) [58] , [59] . Followed by the secondary antibody rat anti-mouse IgG-Alexa Fluor 647 (Invitrogen, 1:200 dilution in M.O.M. diluent) and sections coverslipped with VectaShield with 4′-6-diamidino-2-phenylindole (DAPI; Vector Laboratories). Cultured melanocytes Melan-a (pigmented) and Melan-c (albino) melanocytes were cultured overnight in chamber slides and irradiated with 1.35 kJ m −2 of spectrally defined ultraviolet A (5 min exposure) in PBS. Cells were immediately fixed in cold methanol, rinsed and treated with RNase for 1 h at 37 °C and 8-oxodGuo visualized with N45.1 anti-8-oxodGuo antibody and goat anti-mouse Alexa Fluor 647. Slides were mounted in medium with DAPI and kept at 4 °C until observation with the confocal microscope. Confocal microscopy Low-power images were taken with either Zeiss LSM 710 or 510 confocal systems using Plan Apochromat 20×/0.8. Three fluorescence channels and one transmitted light channel were collected. DAPI was excited with a 405-diode laser and the bandwidth emission filtered between 420–490 nm. Transmitted light images were simultaneously produced by 405 nm line excitation to discriminate melanin but the signal was recorded by a photomultiplier on the forward pathway. The autofluorescence signal was induced by excitation with a 488-nm line of an Argon laser and the emission filtered between 505 and 635 nm. Alexa Fluor 643 was excited by the HeNe 633-nm laser line and the emission filtered with high pass at 650 nm. Images were 1024×1024 pixels with a pixel resolution of 0.439 μm. Confocal images were captured using a pinhole of one Airy unit, providing an optical section thickness of 2.2 μm. High-power confocal images were taken on a Zeiss LSM 710 confocal system using an Axio Examiner Z1 with two standard single-channel photomultipliers and one 32-channel spectral detector (Qazar 34) channel photomultiplier positioned on the backward pathway. A transmitted light photomultiplier was used to record a forward transmitted light image. Confocal images measuring 1024×1024 pixels were taken with an Alpha Plan Apochromat 100×/1.46 (Carl Zeiss) at pixel resolution 0.083 μm. The pinhole was optimized at one Airy unit for Alexa Fluor 647, achieving a confocal section of 0.7 μm. The final confocal image was generated by averaging four scans. To ensure consistent image capturing and standardized conditions, only images taken during one session were compared. Gain and offset of the photomultipliers recording Alexa Fluor 647 were adjusted so that the brightest pixels from the experimental groups only partially filled the image dynamic range. We routinely tested using 32 channels of spectral detection for autofluorescence, derived mainly from skin components but not present in melanocytes. As autofluorescence was much weaker using excitation with 633 nm than with 488 nm, Alexa 637 was chosen to detect immunostaining and 488 nm excitation to generate images of autofluorescence. Image analysis Images were analysed using Volocity (Improvision) and presented with Adobe illustrator. For quantification of nuclear 8-oxodGuo, images of the dermal/epidermal junctional area of the skin taken at ×100 magnification were processed using a protocol created to separate the nuclei based on the DAPI-labelling signal. 8-OxodGuo signal was extracted from the individually identified nuclei as mean pixel intensity. Six to ten fields from replicate or triplicate animals were scored. For some analyses, data from nuclei of pigmented cells only, individually identified by the presence of cytoplasmic melanin from the transmitted light image, were used. For cultured cells, a protocol similar to that for skin sections was followed but replicate ×20 images were used. Quantification of DNA photoproducts by HPLC-MS/MS CPDs and 6-4PPs were quantified by HPLC-MS/MS [23] . Skin from unirradiated or irradiated 3-day-old C57BL/6-HGF or FVB-HGF mice was snap frozen within 10 min of treatment. DNA was extracted and samples injected on an HPLC system (Agilent) connected to a reverse phase HPLC column (150×2 mm 2 ID, 5 μm particle size, ODB, Montluçon, France). Photoproducts were detected by a tandem mass spectrometer (API 3000, SCIEX) [23] . The four CPDs and the four 6-4PPs (TT, TC, CT and CC derivatives) were quantified individually in the same HPLC run as number of lesions per million normal bases. Electron spin resonance Melanin content in mouse dorsal skin was determined using ESR [60] . Characteristic eumelanin and phaeomelanin signals were recorded in liquid nitrogen (77 K) at g =2 in a Bruker EMX spectrometer, which operated in X-band (9.5 GHz) with magnetic field modulation at a frequency of 100 kHz. A mixture (1:1) of 3,4-dihydroxyphenylalanine (DOPA)-melanin and cysteinyl-DOPA-melanin synthesized enzymatically was used as a melanin standard of combined eu- and pheomelanin components, respectively. The spectra of natural and synthetic melanins were recorded at the following instrument parameters: centre field=3,349.1 G, sweep width=120 G, microwave power=68 μW, modulation amplitude=3.00 G, time constant=327.68 ms and conversion time=81.92 ms. An average of 20 scans of each sample was used to determine melanin contents. Reverse transcription (RT)–PCR methods Back skins from unirradiated or irradiated pups were harvested 24 h post irradiation, total RNA extracted and RT–PCR carried out [21] using the following primers: metallothionein 1 (Mt1), forward 5′-CCTCTAAGCGTCACCACGA-3′ and reverse 5′-GCAGGAGCTGGTGCAAGT-3′; endogenous HGF/SF, forward 5′-CCTGACACCACTTGGGAGTA-3′ and reverse 5′-CTTCTCCTTGGCCTTGAATG-3′; and Mt1-HGF/SF transgene, forward 5′-CGACTTCAACGTCCTGAGTACCT-3′ and reverse 5′-GGACCGGCAGAAGTTTGGT-3′. The primers for the endogenous and transgenic HGF/SF were transcript specific, as the primers for endogenous HGF/SF did not detect Mt1-HGF/SF transgenic transcript and vice versa. 18S rRNA (forward 5′-CTTAGAGGGACAAGTGGCG-3′ and reverse 5′-ACGCTGAGCCAGTCAGTGTA-3′) expression was used as the normalizer using the Δ C T method. All primer pairs gave a single PCR product with a single peak in the dissociation curve. The expression data were statistically analysed with two-way ANOVA test, with P <0.05 considered significant. Statistical analysis Kaplan–Meier survival analyses, determination of significance of difference between groups using log-rank test, Students t -test, ANOVA, Mann–Whitney and Kruskal–Wallis rank tests were carried out using Statview (SAS Institute) or SigmaPlot (Systat). The significance of differences between log-transformed slopes was established using Statistxl by ANOVA with Tukey post-hoc tests for multiple comparisons. Tests were two-sided. How to cite this article: Noonan, F.P. et al . Melanoma induction by ultraviolet A but not ultraviolet B radiation requires melanin pigment. Nat. Commun. 3:884 doi: 10.1038/ncomms1893 (2012).